miR-484 regulates mitochondrial network through targeting Fis1 Mitochondria constantly undergo fusion and fission, two necessary processes for the maintenance of organelle fidelity. The abnormal mitochondrial fission participates in the pathogenesis of many diseases, but its regulation remains poorly understood. Here we show that miR-484 can suppress translation of mitochondrial fission protein Fis1, and inhibit Fis1-mediated fission and apoptosis in cardiomyocytes and in the adrenocortical cancer cells. We demonstrate that Fis1 is necessary for mitochondrial fission and apoptosis, and is upregulated during anoxia, whereas miR-484 is downregulated. miR-484 is able to attenuate Fis1 upregulation and mitochondrial fission, by binding to the amino acid coding sequence of Fis1 and inhibiting its translation. In exploring the underlying mechanism of miR-484 downregulation upon apoptosis, we observe that Foxo3a transactivates miR-484 expression. Foxo3a transgenic or knockout mice exhibit, respectively, a high or low level of miR-484 and a reduced or enhanced mitochondrial fission, apoptosis and myocardial infarction. Our data reveal a model of mitochondrial fission regulation by a microRNA. Mitochondria has an important role for the initiation of apoptosis [1] , [2] . Mitochondria constantly undergo fusion and fission that are necessary for the maintenance of organelle fidelity [3] , [4] . Strikingly, most recent studies reveal that abnormal mitochondrial fusion and fission participate in the regulation of apoptosis [5] , [6] . In particular, they are related to a variety of diseases such as skeletal muscle disorders [7] , [8] , [9] , peripheral neuropathy Charcot–Marie–Tooth type 2A [10] , [11] and neurodegeneration [12] . The execution of mitochondrial fission in mammalian cells requires the participation of a large number of proteins [13] . For example, dynamin-related protein-1 (Drp1) is involved in the initiation of mitochondrial fission [3] . Mitofusin-1 (Mfn-1) controls mitochondrial fusion [14] and it can prevent mitochondrial fission [15] . Bax/Bak promotes sumoylation of Drp1 and its stable association with mitochondria during apoptosis [16] . Thus, mitochondrial fission is regulated by a complex interplay of proteins. Foxo3a is a transcription factor and can either initiate or inhibit apoptosis, depending on the cell types and the cellular contexts. It can provoke apoptosis in haematopoietic [17] and neuronal cells [18] , but prevent apoptosis in neutrophils [19] . Hitherto, it is not yet clear whether Foxo3a is a component in the cascades of mitochondrial fission programme. Fis1 is a protein that is involved in mitochondrial fission of mammalian cells [20] . It is exclusively localized to mitochondria [21] and expressed at low levels under physiological condition. However, it can be upregulated during apoptosis, and modulation of Fis1 levels affects apoptotic progress [22] . It remains to be elucidated how Fis1 expression is regulated under pathophysiological condition. MicroRNAs (miRNAs) act as negative regulators of gene expression [23] , [24] , [25] , [26] , [27] , [28] , [29] . Strikingly, a single miRNA is even able to modulate complex physiological or disease phenotypes by regulating the entire functional networks [26] , [30] , [31] . Apoptosis can be regulated by miRNAs. Some miRNAs participate in the initiation of apoptosis. For example, miR-122 modulates cyclin G1 silencing and increases sensitivity of cells to undergoing apoptosis [32] . The miR-23a-27a-24-2 cluster induces caspase-dependent and -independent apoptosis [33] . Histone deacetylases are related to cell survival and their expression can be repressed by miR-449a [34] . There are also miRNAs that can inhibit apoptosis. miR-206 prevents apoptosis by targeting notch3 [35] . The miR-17-92 cluster is a novel target for p53-mediated transcriptional repression [36] . In addition, p53 is also regulated by miR-125b [37] . Our present study shows that miR-484 can repress Fis1 expression and is able to inhibit mitochondrial fission through targeting Fis1. Strikingly, miR-484 binds to the amino acid coding region of Fis1. miR-484 is downregulated in response to apoptotic stimulation. In exploring the mechanism by which miR-484 expression is regulated, we observed that Foxo3a can transactivate miR-484 expression. Foxo3a inhibits Fis1 expression and the consequent mitochondrial fission through transcriptionally targeting miR-484. We found that the regulation of miR-484 on Fis1 not only occurs in the heart, but also in the cancer cells. Our results reveal a mitochondrial fission-regulating model, which is composed of Foxo3a, miR-484 and Fis1. Fis1 regulates mitochondrial fission and apoptosis We tested the role of Fis1 in mitochondrial dynamics in cardiomyocytes and myocardial infarction. Anoxia could induce mitochondrial fission ( Supplementary Fig. S1a ) with an elevated protein level of Fis1 ( Supplementary Fig. S1b ). Knockdown of Fis1 attenuated mitochondrial fission and apoptosis ( Fig. 1a and Supplementary Fig. S1c ). Anoxia induced an alteration in the expression of Drp1, mitochondial fission factor (MFF), Mfn 1, Mfn 2 and optic atrophy type I (Opa1), which was not affected by Fis1 small interfering RNA ( Supplementary Fig. S1d ). Enforced expression of Fis1 led to mitochondrial fission and apoptosis ( Supplementary Fig. S2a ). We tested whether Fis1 has a role in the pathogenesis of myocardial infarction. Upon ischaemia/reperfusion (I/R), knockdown of Fis1 attenuated mitochondrial fission and apoptosis ( Fig. 1b and Supplementary Fig. S2b ). Further, Fis1 knockdown reduced myocardial infarction sizes revealed by morphometric analysis (upper panels, Fig. 1c ) and quantification (lower panel, Fig. 1c ). These data suggest that Fis1 participates in mediating the signal for mitochondrial fission and apoptosis in the heart. 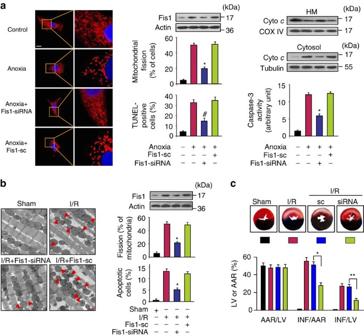Figure 1: Fis1 regulates mitochondrial fission and apoptosis. (a) Knockdown of Fis1 inhibits mitochondrial fission induced by anoxia. Cardiomyocytes were infected with adenoviral Fis1-small interfering RNA (siRNA) or its scramble form (sc), and then exposed to anoxia. Left panel: mitochondria were visualized by staining with MitoTracker Red. Scale bar equals 10 μm. Middle panel: counting of cells with mitochondrial fission and apoptosis. Fis1 levels were analysed by immunoblot. The results are expressed as mean±s.e.m. of three independent experiments. *P<0.001 versus anoxia alone;#P<0.01 versus anoxia alone. Data were statistically analysed by one-way analysis of variance (ANOVA). Right panel: cytochrome c (Cyto c) distributions in mitochondria-enriched heavy membranes (HM) or cytosol detected by immunoblot and caspase-3 activity analysis. The results are expressed as mean±s.e.m. of four independent experiments. *P<0.001 versus anoxia alone. Data were statistically analysed by one-way ANOVA. (b) Fis1 is necessary for mitochondrial fission upon I/R. Intracoronary delivery of adenoviral constructs of Fis1 siRNA or its scramble form (sc) to the hearts was described in the section ofSupplementary Methods. Mice were subjected to 45 min ischaemia and 3 h reperfusion. Thin-section electron micrographs from the sham or ischaemic hearts were assessed by electron microscopy (EM). Representative EM images of hearts were shown in left panel. Scale bar equals 1 μm. The arrows indicate fission mitochondria. Counting of fragmented mitochondria and apoptosis, and Fis1 levels analysed by immunoblot are shown in the right panel.n=15 slices from five animals. *P<0.001 versus I/R alone. Data were statistically analysed by one-way ANOVA. (c) Fis1 participates in the induction of myocardial infarction. Mice were treated as described in (b). The upper panels are representative photos of midventricular myocardial slices. The heart section from the group of I/R alone showed infarcted myocardium (white) in the risk region (white plus red). The heart section from the group of I/R plus siRNA showed less infarction. The lower panel shows infarct sizes.n=five animals. *P<0.001, **P<0.05. Data were statistically analysed by one-way ANOVA. Figure 1: Fis1 regulates mitochondrial fission and apoptosis. ( a ) Knockdown of Fis1 inhibits mitochondrial fission induced by anoxia. Cardiomyocytes were infected with adenoviral Fis1-small interfering RNA (siRNA) or its scramble form (sc), and then exposed to anoxia. Left panel: mitochondria were visualized by staining with MitoTracker Red. Scale bar equals 10 μm. Middle panel: counting of cells with mitochondrial fission and apoptosis. Fis1 levels were analysed by immunoblot. The results are expressed as mean±s.e.m. of three independent experiments. * P <0.001 versus anoxia alone; # P <0.01 versus anoxia alone. Data were statistically analysed by one-way analysis of variance (ANOVA). Right panel: cytochrome c (Cyto c) distributions in mitochondria-enriched heavy membranes (HM) or cytosol detected by immunoblot and caspase-3 activity analysis. The results are expressed as mean±s.e.m. of four independent experiments. * P <0.001 versus anoxia alone. Data were statistically analysed by one-way ANOVA. ( b ) Fis1 is necessary for mitochondrial fission upon I/R. Intracoronary delivery of adenoviral constructs of Fis1 siRNA or its scramble form (sc) to the hearts was described in the section of Supplementary Methods . Mice were subjected to 45 min ischaemia and 3 h reperfusion. Thin-section electron micrographs from the sham or ischaemic hearts were assessed by electron microscopy (EM). Representative EM images of hearts were shown in left panel. Scale bar equals 1 μm. The arrows indicate fission mitochondria. Counting of fragmented mitochondria and apoptosis, and Fis1 levels analysed by immunoblot are shown in the right panel. n =15 slices from five animals. * P <0.001 versus I/R alone. Data were statistically analysed by one-way ANOVA. ( c ) Fis1 participates in the induction of myocardial infarction. Mice were treated as described in ( b ). The upper panels are representative photos of midventricular myocardial slices. The heart section from the group of I/R alone showed infarcted myocardium (white) in the risk region (white plus red). The heart section from the group of I/R plus siRNA showed less infarction. The lower panel shows infarct sizes. n =five animals. * P <0.001, ** P <0.05. Data were statistically analysed by one-way ANOVA. Full size image miR-484 targets the amino acid coding sequence of Fis1 miRNA is able to suppress gene expression. To explore the underlying mechanism by which Fis1 is upregulated, we tested whether miRNA can control Fis1 expression. miR-484 is a cardiac-abundant miRNA [38] , but was downregulated upon anoxia ( Supplementary Fig. S3a ) and ischaemia ( Supplementary Fig. S3b ). We tested whether miR-484 is related to Fis1 expression. Enforced expression of miR-484 could reduce Fis1 levels ( Fig. 2a ). Knockdown of endogenous miR-484 resulted in an elevation of Fis1 levels ( Supplementary Fig. S3c ). The miR-484 transgenic mice demonstrated a reduced Fis1 level in response to I/R ( Fig. 2b ). 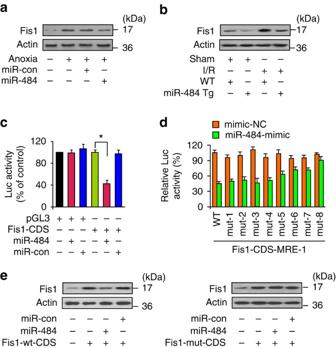Figure 2: miR-484 targets the amino acid coding sequence of Fis1. (a) Forced expression of miR-484 attenuates the increase in Fis1 levels upon anoxia. Cardiomyocytes were infected with adenoviral miR-484 or miR-484 control (miR-con). After 24 h of infection, cells were exposed to anoxia and harvested 1 h after treatment for the analysis of Fis1 by immunoblot. (b) miR-484 transgenic mice attenuate the increase in Fis1 levels upon I/R. miR-484 transgenic mice (miR-484 Tg) or wild-type mice (WT) were subjected to 45 min ischaemia and 3 h reperfusion, and Fis1 levels were detected by immunoblot. (c) miR-484 suppresses Fis1 translation. HEK293 cells were transfected with the luciferase constructs of the Fis1-CDS, along with the expression plasmids for miR-484 or miR-con. The results are expressed as mean±s.e.m. of three independent experiments. *P<0.001. Data were statistically analysed by one-way analysis of variance. (d) Luciferase assays of mutated MREs. Luciferase results for co-transfection of miR-484 mimic or mimic-negative control (mimic-NC) with various luciferase-MRE mutants. The data are expressed as the relative levels to WT or the eight mutants in the absence of mimic or mimic-NC, respectively. The results are expressed as mean±s.e.m. of three independent experiments. (e) miR-484 can suppress the expression of Fis1 with WT, but not mutated CDS. Cardiomyocytes were co-infected with the adenoviral miR-484, or its control form (miR-con), along with Fis1 with WT CDS (Fis1-wt-CDS) or the mutated CDS (Fis1-mut-CDS, which has the same mutations as CDS-mut-8) at a multiplicity of infection of 100. Fis1 levels were detected by immunoblot. Figure 2: miR-484 targets the amino acid coding sequence of Fis1. ( a ) Forced expression of miR-484 attenuates the increase in Fis1 levels upon anoxia. Cardiomyocytes were infected with adenoviral miR-484 or miR-484 control (miR-con). After 24 h of infection, cells were exposed to anoxia and harvested 1 h after treatment for the analysis of Fis1 by immunoblot. ( b ) miR-484 transgenic mice attenuate the increase in Fis1 levels upon I/R. miR-484 transgenic mice (miR-484 Tg) or wild-type mice (WT) were subjected to 45 min ischaemia and 3 h reperfusion, and Fis1 levels were detected by immunoblot. ( c ) miR-484 suppresses Fis1 translation. HEK293 cells were transfected with the luciferase constructs of the Fis1-CDS, along with the expression plasmids for miR-484 or miR-con. The results are expressed as mean±s.e.m. of three independent experiments. * P <0.001. Data were statistically analysed by one-way analysis of variance. ( d ) Luciferase assays of mutated MREs. Luciferase results for co-transfection of miR-484 mimic or mimic-negative control (mimic-NC) with various luciferase-MRE mutants. The data are expressed as the relative levels to WT or the eight mutants in the absence of mimic or mimic-NC, respectively. The results are expressed as mean±s.e.m. of three independent experiments. ( e ) miR-484 can suppress the expression of Fis1 with WT, but not mutated CDS. Cardiomyocytes were co-infected with the adenoviral miR-484, or its control form (miR-con), along with Fis1 with WT CDS (Fis1-wt-CDS) or the mutated CDS (Fis1-mut-CDS, which has the same mutations as CDS-mut-8) at a multiplicity of infection of 100. Fis1 levels were detected by immunoblot. Full size image To understand whether miR-484 regulates Fis1 through a direct or indirect manner, we analysed the 3′-untranslated region (UTR) sequence of Fis1; there is no highly conserved complementary sequence of miR-484. We analysed the coding region of rat Fis1 and observed that it contains the complementary sequence of miR-484, which is evolutionarily conserved ( Supplementary Fig. S4 ). The luciferase reporter assay revealed that miR-484 could reduce Fis1 translation ( Fig. 2c ). Introduction of mutations that disrupt base pairing between miR-484 and Fis1 ( Supplementary Fig. S5c ) rescued luciferase expression ( Fig. 2d ) and Fis1 protein expression ( Fig. 2e ), indicating that the recognition of miR-484 to Fis1 coding sequence (CDS) region is specific. miR-484 regulates mitochondrial fission and apoptosis Subsequently, we tested whether miR-484 has a functional role in the heart. In the cellular model, enforced expression of miR-484 inhibited mitochondrial fission and apoptosis upon anoxia ( Fig. 3a ). In the animal model, miR-484 transgenic mice exhibited attenuated mitochondrial fission and apoptosis ( Supplementary Fig. S6a,b ). To understand the role of endogenous miR-484, we employed the antagomir of miR-484 to knockdown endogenous miR-484 ( Supplementary Fig. S7a,b ). Administration of miR-484 antagomir could potentiate mitochondrial fission and apoptotic response ( Supplementary Fig. S7c ) and enlarge myocardial infarction sizes ( Supplementary Fig. S7d ). Taken together, it appears that miR-484 is able to prevent mitochondrial fission, apoptosis and myocardial infarction in the heart. 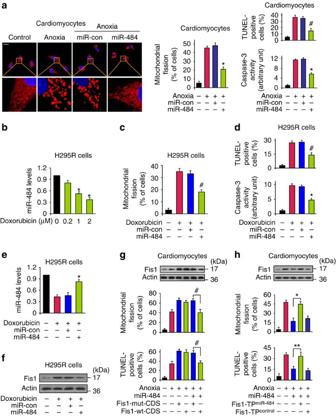Figure 3: miR-484 regulates mitochondrial fission and apoptosis in the heart and in cancer cells. (a) miR-484 prevents mitochondrial fission and apoptosis. Cardiomyocytes were infected with adenoviral miR-484 or its control (miR-con). Scale bar equals 20 μm. The results are expressed as mean±s.e.m. of three (mitochondrial fission, TUNEL (terminal deoxynucleotidyl transferase dUTP nick end labelling)) or four (caspase-3 activity) independent experiments. *P<0.001 versus anoxia alone;#P<0.01 versus anoxia alone. Data were statistically analysed by one-way analysis of variance (ANOVA). (b) Doxorubicin induces a reduction in miR-484 levels in H295R cells. The results are expressed as mean±s.e.m. of three independent experiments. *P<0.001 versus control. Data were statistically analysed by Student'st-test. (c,d) miR-484 inhibits mitochondrial fission and apoptosis. H295R were infected with adenoviral miR-484 or its control (miR-con). Mitochondrial fission (c) and apoptosis (d) were analysed. The results are expressed as mean±s.e.m. of three (mitochondrial fission, TUNEL) or four (caspase-3 activity) independent experiments.#P<0.01 versus doxorubicin alone; *P<0.001 versus doxorubicin alone. Data were statistically analysed by one-way ANOVA. (e) Analysis of miR-484 levels. Cells were treated as described for (c), miR-484 levels were detected by qRT–PCR. The results are expressed as mean±s.e.m. of three independent experiments. *P<0.001 versus doxorubicin alone. Data were statistically analysed by one-way ANOVA. (f) Analysis of Fis1 levels. Cells were treated as described for (c). (g) miR-484 can attenuate Fis1 levels, mitochondrial fission and apoptosis in the presence of Fis1 with wild-type CDS (Fis1-wt-CDS), but not its mutated form (Fis1-mut-CDS). Cardiomyocytes were infected with the adenoviral miR-484, along with the constructs of Fis1-wt-CDS or Fis1-mut-CDS at a multiplicity of infection of 50. The results are expressed as mean±s.e.m. of three independent experiments.#P<0.01. Data were statistically analysed by one-way ANOVA. (h) Fis1 target protector reduces the inhibitory effect of miR-484 on mitochondrial fission and apoptosis. Cardiomyocytes were infected with adenoviral miR-484, transfected with the target protector (Fis1-TPmiR-484) or the control (Fis1-TPcontrol). Fis1 was analysed by immunoblot (upper panel). The results are expressed as mean±s.e.m. of three independent experiments. *P<0.001, **P<0.05. Data were statistically analysed by one-way ANOVA. Figure 3: miR-484 regulates mitochondrial fission and apoptosis in the heart and in cancer cells. ( a ) miR-484 prevents mitochondrial fission and apoptosis. Cardiomyocytes were infected with adenoviral miR-484 or its control (miR-con). Scale bar equals 20 μm. The results are expressed as mean±s.e.m. of three (mitochondrial fission, TUNEL (terminal deoxynucleotidyl transferase dUTP nick end labelling)) or four (caspase-3 activity) independent experiments. * P <0.001 versus anoxia alone; # P <0.01 versus anoxia alone. Data were statistically analysed by one-way analysis of variance (ANOVA). ( b ) Doxorubicin induces a reduction in miR-484 levels in H295R cells. The results are expressed as mean±s.e.m. of three independent experiments. * P <0.001 versus control. Data were statistically analysed by Student's t -test. ( c , d ) miR-484 inhibits mitochondrial fission and apoptosis. H295R were infected with adenoviral miR-484 or its control (miR-con). Mitochondrial fission ( c ) and apoptosis ( d ) were analysed. The results are expressed as mean±s.e.m. of three (mitochondrial fission, TUNEL) or four (caspase-3 activity) independent experiments. # P <0.01 versus doxorubicin alone; * P <0.001 versus doxorubicin alone. Data were statistically analysed by one-way ANOVA. ( e ) Analysis of miR-484 levels. Cells were treated as described for ( c ), miR-484 levels were detected by qRT–PCR. The results are expressed as mean±s.e.m. of three independent experiments. * P <0.001 versus doxorubicin alone. Data were statistically analysed by one-way ANOVA. ( f ) Analysis of Fis1 levels. Cells were treated as described for ( c ). ( g ) miR-484 can attenuate Fis1 levels, mitochondrial fission and apoptosis in the presence of Fis1 with wild-type CDS (Fis1-wt-CDS), but not its mutated form (Fis1-mut-CDS). Cardiomyocytes were infected with the adenoviral miR-484, along with the constructs of Fis1-wt-CDS or Fis1-mut-CDS at a multiplicity of infection of 50. The results are expressed as mean±s.e.m. of three independent experiments. # P <0.01. Data were statistically analysed by one-way ANOVA. ( h ) Fis1 target protector reduces the inhibitory effect of miR-484 on mitochondrial fission and apoptosis. Cardiomyocytes were infected with adenoviral miR-484, transfected with the target protector (Fis1-TP miR-484 ) or the control (Fis1-TP control ). Fis1 was analysed by immunoblot (upper panel). The results are expressed as mean±s.e.m. of three independent experiments. * P <0.001, ** P <0.05. Data were statistically analysed by one-way ANOVA. Full size image We attempted to understand whether the regulation of miR-484 on Fis1 is cell-type specific. It has been reported that miR-484 is upregulated in massive macronodular adrenocortical disease [39] . We thus tested whether miR-484 has a functional role in adrenocortical cancer cells. We treated the cells with doxorubicin and observed that miR-484 levels were decreased in cells treated with higher doses of doxorubicin ( Fig. 3b ). Doxorubicin was able to induce mitochondrial fission ( Fig. 3c ) as well as apoptosis ( Fig. 3d ), and this effect was counteracted by enforced expression of miR-484. miR-484 levels were higher in cells expressing exogenous miR-484 and treated with doxorubicin ( Fig. 3e ). Concomitantly, miR-484 could affect Fis1 levels ( Fig. 3f ). These data suggest that the axis of miR-484 and Fis1 functionally controls mitochondrial fission programme in adrenocortical cancer cells. We explored how miR-484 exerts its effect on the mitochondrial network. As miR-484 is able to suppress Fis1 expression, we thus tested whether Fis1 is a mediator of miR-484. Although miR-484 could inhibit mitochondrial fission and apoptosis, this inhibitory effect was significantly abolished by Fis1 with mutated coding sequence, but not the wild-type Fis1 ( Fig. 3g ). To confirm the relationship between miR-484 and Fis1 in mitochondrial fission machinery, we employed the target protector technology in which a target protector is able to disrupt the specific interaction of miRNA–mRNA pairs [40] . To this end, we produced Fis1 target protector and observed that the inhibitory effect of miR-484 on mitochondrial fission and apoptosis was reduced in the presence of Fis1 target protector ( Fig. 3h ). These data suggest that miR-484 targets Fis1 in the cascades of mitochondrial fission and apoptosis. Foxo3a transactivates miR-484 We asked why miR-484 is downregulated in response to the pathological insults. Our previous work has shown that the expression of a miRNA can be regulated at the transcriptional level [41] . We analysed the promoter region of rat miR-484 and observed that there is an optimal consensus-binding site of Foxo3a ( Fig. 4a ), and there are also binding sites in the promoter regions of human and mouse miR-484 ( Supplementary Fig. S8a ). We tested whether Foxo3a can bind to the promoter region of miR-484. The chromatin immunoprecipitation (ChIP)–quantitative PCR (qPCR) assay revealed that Foxo3a bound to the miR-484 promoter under the physiological condition. Anoxic treatment led to a reduction in the association levels of Foxo3a with the miR-484 promoter ( Fig. 4b ). The luciferase assay demonstrated that the constitutively active Foxo3a (caFoxo3a) stimulated the miR-484 promoter activity ( Fig. 4c ). Anoxia induced a reduction in Foxo3a expression levels ( Supplementary Fig. S8b ) and miR-484 promoter activity ( Fig. 4d ). Foxo3a was decreased upon doxorubicin treatment ( Supplementary Fig. S8c ). Enforced expression of caFoxo3a led to an elevation of miR-484 levels ( Fig. 4e ). The decrease of miR-484 induced by anoxia was attenuated by caFoxo3a ( Fig. 4f ). Knockdown of Foxo3a induced a decrease in miR-484 expression levels ( Fig. 4g ). The caFoxo3a transgenic mice demonstrated a higher level of miR-484 ( Fig. 4h ), whereas Foxo3a knockout (KO) mice exhibited a low level of miR-484 ( Fig. 4i ). These data suggest that Foxo3a can transcriptionally upregulate miR-484. 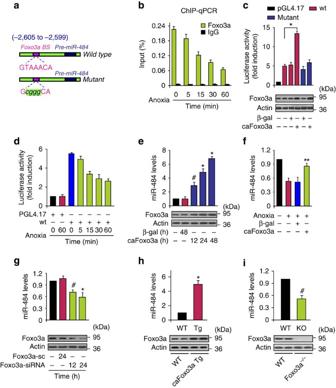Figure 4: Foxo3a transactivates miR-484. (a) Rat miR-484 promoter region contains a potential Foxo3a-binding site. (b) ChIP–qPCR analysis of Foxo3a binding to the promoter of miR-484. The results are expressed as mean±s.e.m. of three independent experiments. (c) Foxo3a activates miR-484 promoter activity. Cardiomyocytes were treated with the adenoviral β-gal or caFoxo3a, the constructs of the empty vector (pGL-4.17), the wild-type promoter (wt) or the promoter with mutations in the binding site (mutant), respectively. The results are expressed as mean±s.e.m. of three independent experiments. *P<0.001. Data were statistically analysed by one-way analysis of variance (ANOVA). (d) Anoxia induces a reduction of miR-484 promoter activity. Cardiomyocytes were transfected with wt or empty vector (pGL-4.17). The results are expressed as mean±s.e.m. of three independent experiments. (e) Foxo3a stimulates miR-484 expression. Cardiomyocytes were infected with adenoviral β-gal or caFoxo3a at a multiplicity of infection (MOI) of 50. The results are expressed as mean±s.e.m. of three independent experiments. *P<0.001 versus control;#P<0.01 versus control. Data were statistically analysed by Student'st-test. (f) caFoxo3a attenuates the decrease of miR-484. Cardiomyocytes were infected with adenoviral β-gal or caFoxo3a at an MOI of 50. The results are expressed as mean±s.e.m. of three independent experiments. **P<0.05 versus anoxia alone. Data were statistically analysed by one-way ANOVA. (g) Knockdown of endogenous Foxo3a leads to a reduction in miR-484 levels. Cardiomyocytes were infected with adenoviral Foxo3a-siRNA or its scramble form (Foxo3a-sc) at an MOI of 100. The results are expressed as mean±s.e.m. of three independent experiments. *P<0.001 versus control.#P<0.01 versus control. Data were statistically analysed by Student'st-test. (h) miR-484 levels in caFoxo3a transgenic mice (Tg). qRT–PCR and immunoblot were performed with caFoxo3a Tg or the wild-type mice (WT).n=18 from 6 animals. *P<0.001 versus WT. Data were statistically analysed by Student'st-test. (i) miR-484 levels in Foxo3a-deficient mice. Foxo3a KO mice, WT littermates.n=18 from 6 animals.#P<0.01 versus WT. Data were statistically analysed by Student'st-test. Figure 4: Foxo3a transactivates miR-484. ( a ) Rat miR-484 promoter region contains a potential Foxo3a-binding site. ( b ) ChIP–qPCR analysis of Foxo3a binding to the promoter of miR-484. The results are expressed as mean±s.e.m. of three independent experiments. ( c ) Foxo3a activates miR-484 promoter activity. Cardiomyocytes were treated with the adenoviral β-gal or caFoxo3a, the constructs of the empty vector (pGL-4.17), the wild-type promoter (wt) or the promoter with mutations in the binding site (mutant), respectively. The results are expressed as mean±s.e.m. of three independent experiments. * P <0.001. Data were statistically analysed by one-way analysis of variance (ANOVA). ( d ) Anoxia induces a reduction of miR-484 promoter activity. Cardiomyocytes were transfected with wt or empty vector (pGL-4.17). The results are expressed as mean±s.e.m. of three independent experiments. ( e ) Foxo3a stimulates miR-484 expression. Cardiomyocytes were infected with adenoviral β-gal or caFoxo3a at a multiplicity of infection (MOI) of 50. The results are expressed as mean±s.e.m. of three independent experiments. * P <0.001 versus control; # P <0.01 versus control. Data were statistically analysed by Student's t -test. ( f ) caFoxo3a attenuates the decrease of miR-484. Cardiomyocytes were infected with adenoviral β-gal or caFoxo3a at an MOI of 50. The results are expressed as mean±s.e.m. of three independent experiments. ** P <0.05 versus anoxia alone. Data were statistically analysed by one-way ANOVA. ( g ) Knockdown of endogenous Foxo3a leads to a reduction in miR-484 levels. Cardiomyocytes were infected with adenoviral Foxo3a-siRNA or its scramble form (Foxo3a-sc) at an MOI of 100. The results are expressed as mean±s.e.m. of three independent experiments. * P <0.001 versus control. # P <0.01 versus control. Data were statistically analysed by Student's t -test. ( h ) miR-484 levels in caFoxo3a transgenic mice (Tg). qRT–PCR and immunoblot were performed with caFoxo3a Tg or the wild-type mice (WT). n =18 from 6 animals. * P <0.001 versus WT. Data were statistically analysed by Student's t -test. ( i ) miR-484 levels in Foxo3a-deficient mice. Foxo3a KO mice, WT littermates. n =18 from 6 animals. # P <0.01 versus WT. Data were statistically analysed by Student's t -test. Full size image Foxo3a inhibits mitochondrial fission through miR-484 and Fis1 We tested the role of Foxo3a in mitochondrial fission and apoptosis. Anoxia-induced mitochondrial fission and apoptosis were attenuated by caFoxo3a ( Fig. 5a ). The caFoxo3a transgenic mice exhibited a reduced level of mitochondrial fission ( Fig. 5b ), apoptosis ( Fig. 5c ) and myocardial infarction sizes ( Fig. 5d ). Thus, Foxo3a is able to inhibit mitochondrial fission and apoptosis in the heart. 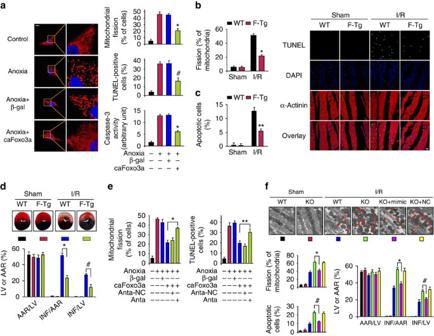Figure 5: Foxo3a inhibits mitochondrial fission through miR-484 and Fis1. (a) Foxo3a inhibits mitochondrial fission and apoptosis. Cardiomyocytes were infected with adenoviral caFoxo3a or β-gal. Scale bar equals 10 μm. The results are expressed as mean±s.e.m. of three (mitochondrial fission, TUNEL (terminal deoxynucleotidyl transferase dUTP nick end labelling)) or four (caspase-3 activity) independent experiments. *P<0.001 versus anoxia alone;#P<0.01 versus anoxia alone. Data were statistically analysed by one-way analysis of variance (ANOVA). (b) Mitochondrial fission was reduced in caFoxo3a transgenic mice upon I/R. caFoxo3a transgenic mice (F-Tg) or wild-type mice (WT) were subjected to I/R, and mitochondrial fission was analysed.n=15 slices from five animals. *P<0.001 versus WT+I/R. Data were statistically analysed by Student'st-test. (c) caFoxo3a Tg mice exhibit less apoptosis upon I/R. Right panel shows representative images of ventricular myocardium sections from WT and F-Tg mice.n=15 slices from five animals. **P<0.05 versus WT+I/R. Data were statistically analysed by Student'st-test. (d) F-Tg are resistant to undergo myocardial infarction induced by I/R. F-Tg and WT mice were exposed to I/R. The upper panels are representative photos of midventricular myocardial slices. The lower panel shows infarct sizes.n=five animals. *P<0.001;#P<0.01. Data were statistically analysed by Student'st-test. (e) Knockdown of miR-484 leads to the attenuation of caFoxo3a inhibitory effect on mitochondrial fission and apoptosis. Cardiomyocytes were infected with adenoviral caFoxo3a or β-gal, transfected with miR-484 antagomir (Anta) or antagomir-negative control (Anta-NC). The results are expressed as mean±s.e.m. of three independent experiments. *P<0.001. **P<0.05. Data were statistically analysed by one-way ANOVA. (f) miR-484 reduces mitochondrial fission, apoptosis and myocardial infarction in Foxo3a KO mice. Foxo3a KO mice were administrated with miR-484 mimic or mimic-negative control (NC), and then exposed to I/R together with WT mice. The arrows indicate fission mitochondria. Scale bar equals 1 μm. Mitochondrial fission, apoptosis and infarct sizes are shown in lower panels.n=15 slices from five animals. *P<0.001;#P<0.01. Data were statistically analysed by one-way ANOVA. Figure 5: Foxo3a inhibits mitochondrial fission through miR-484 and Fis1. ( a ) Foxo3a inhibits mitochondrial fission and apoptosis. Cardiomyocytes were infected with adenoviral caFoxo3a or β-gal. Scale bar equals 10 μm. The results are expressed as mean±s.e.m. of three (mitochondrial fission, TUNEL (terminal deoxynucleotidyl transferase dUTP nick end labelling)) or four (caspase-3 activity) independent experiments. * P <0.001 versus anoxia alone; # P <0.01 versus anoxia alone. Data were statistically analysed by one-way analysis of variance (ANOVA). ( b ) Mitochondrial fission was reduced in caFoxo3a transgenic mice upon I/R. caFoxo3a transgenic mice (F-Tg) or wild-type mice (WT) were subjected to I/R, and mitochondrial fission was analysed. n =15 slices from five animals. * P <0.001 versus WT+I/R. Data were statistically analysed by Student's t -test. ( c ) caFoxo3a Tg mice exhibit less apoptosis upon I/R. Right panel shows representative images of ventricular myocardium sections from WT and F-Tg mice. n =15 slices from five animals. ** P <0.05 versus WT+I/R. Data were statistically analysed by Student's t -test. ( d ) F-Tg are resistant to undergo myocardial infarction induced by I/R. F-Tg and WT mice were exposed to I/R. The upper panels are representative photos of midventricular myocardial slices. The lower panel shows infarct sizes. n =five animals. * P <0.001; # P <0.01. Data were statistically analysed by Student's t -test. ( e ) Knockdown of miR-484 leads to the attenuation of caFoxo3a inhibitory effect on mitochondrial fission and apoptosis. Cardiomyocytes were infected with adenoviral caFoxo3a or β-gal, transfected with miR-484 antagomir (Anta) or antagomir-negative control (Anta-NC). The results are expressed as mean±s.e.m. of three independent experiments. * P <0.001. ** P <0.05. Data were statistically analysed by one-way ANOVA. ( f ) miR-484 reduces mitochondrial fission, apoptosis and myocardial infarction in Foxo3a KO mice. Foxo3a KO mice were administrated with miR-484 mimic or mimic-negative control (NC), and then exposed to I/R together with WT mice. The arrows indicate fission mitochondria. Scale bar equals 1 μm. Mitochondrial fission, apoptosis and infarct sizes are shown in lower panels. n =15 slices from five animals. * P <0.001; # P <0.01. Data were statistically analysed by one-way ANOVA. Full size image The regulation of Foxo3a on miR-484 expression led us to consider whether these two molecules are functionally related in regulating mitochondrial dynamics and apoptosis. Knockdown of miR-484 led to the attenuation of caFoxo3a inhibitory effect on mitochondrial fission and apoptosis induced by anoxia ( Fig. 5e ). To further understand the physiological significance of Foxo3a-miR-484 axis in the heart, we employed Foxo3a KO mice. In response to I/R, Foxo3a-deficient mice demonstrated more mitochondrial fission and apoptosis, as well as an enlarged myocardial infarction size. miR-484 mimic ( Supplementary Fig. S9a,b ) reduced mitochondrial fission, apoptosis and myocardial infarction sizes in Foxo3a-deficient mice ( Fig. 5f ). These data suggest that miR-484 can influence the effect of Foxo3a. We tested whether Foxo3a-miR-484 axis is related to Fis1 expression. caFoxo3a led to a reduction of Fis1 levels upon anoxic treatment, but knockdown of miR-484 was able to abolish the effect of caFoxo3a on Fis1 expression ( Supplementary Fig. S9c ). A variety of Foxo3a downstream mediators have been identified. We attempted to understand whether other downstream mediators of Foxo3a are involved in the fission and apoptotic programme. Catalase can be regulated by Foxo3a [42] ; we thus tested whether it can affect mitochondrial fission. Catalase suppressed mitochondrial fission and apoptosis ( Supplementary Fig. S10a ). The heart contains many miRNAs. It is necessary to know if other miRNAs can affect apoptosis. We tested whether miR-21 is able to influence apoptosis upon anoxia. Anoxia induced a reduction of miR-21, and overexpression of miR-21 attenuated apoptosis ( Supplementary Fig. S10b ). Cardiac fibroblasts and cardiomyocytes have a distinct character. We detected the mitochondrial morphology of cardiac fibroblasts when Fis1 is depleted. Knockdown of Fis1 attenuated apoptosis, but not mitochondrial fission ( Supplementary Fig. S10c ), suggesting that different types of cells may require differential factors to trigger fission programme. Taken together, Foxo3a and miR-484 constitute an axis regulating mitochondrial dynamics and apoptosis in the heart. Our present study revealed that miR-484 can repress Fis1 expression and inhibit mitochondrial fission through targeting Fis1. miRNAs can bind to the 3′-UTR of mRNAs [43] . Our work demonstrated that miR-484 regulates Fis1 through targeting the amino acid coding sequence. Noticeably, Foxo3a can inhibit apoptosis [19] , [44] . In consistence with the anti-apoptotic function of Foxo3a, we identified that Foxo3a can transactivate miR-484 expression. Foxo3a inhibits Fis1 expression and the consequent mitochondrial fission through transcriptionally targeting miR-484. Our results reveal a novel regulatory model of mitochondrial fission by miRNA and Foxo3a. In most cases, miRNAs are reported to bind to the 3′-UTR of mRNAs, thereby inhibiting mRNA translation or promoting mRNA degradation [43] . Our present study revealed that miR-484 can repress Fis1 expression through targeting its amino acid coding sequence rather than its 3′-UTR. This is in consistence with the most recent work demonstrating that miRNAs can interact with the coding region of mRNA [45] , [46] . For example, miR-148 represses DNA methyltransferase 3b gene expression through a region in its coding sequence [47] . Strikingly, we found that the binding sites of miR-484 in the amino acid coding sequences of Fis1 are evolutionarily conserved in many species, including human, rat and mouse. In particular, our results have demonstrated that the regulation of miR-484 on Fis1 occurs not only in rat and mouse models, but also in human cancer cells. Foxo3a is known to be able to trigger apoptotic programme [18] . Nevertheless, there are also reports showing that it can inhibit apoptosis [19] , [44] . It stimulates the expression of the anti-apoptotic factors including manganese superoxide dismutase [48] and catalase [49] . Our present work unveils that Foxo3a can transactivate miR-484 expression. Foxo3a inhibits Fis1 expression and the consequent mitochondrial fission through transcriptionally targeting miR-484. Our work further demonstrated that Foxo3a transgenic mice exhibited resistance to undergoing myocardial infarction. These results suggest that Foxo3a has a cardiac protective role, and miR-484 is a mediator to convey its function against mitochondrial fission and apoptosis. The decreased cell death is related to tumourigenesis and tumour resistance to chemotherapy. Unfortunately, a major obstacle of chemotherapy for tumour is the cardiac toxicity due to apoptosis. Our present study reveals that miR-484 and Fis1 constitute an axis controlling mitochondrial connectivity and apoptosis in both the heart and cancer. Our results suggest that miR-484 and Fis1 can be targets for developing specific mitochondria-targeting cardioprotective drugs, as well as tumour-specific mitochondrial toxic agents. Growing evidence has revealed that the mitochondrial fusion and fission programme is regulated by a large number of proteins, such as Fis1, MFF, Mfn 1, Mfn 2, Drp1, Opa1, mitochondrial ubiquitin ligase, mitochondrial protein 18 kDa, Pink 1, Parkin, and so on [50] . These proteins have an important role in a variety of fields, such as neurobiology, heart, cancers and kidney. Indeed, our results indicate that the regulation of miR-484 on Fis1 occurs not only in the heart, but also in the cancer cells. Our results are consistent with a recent report that shows the important role of Fis1 in conveying the apoptotic signal [51] . Fis1 and Bap31 form a complex that spans the mitochondria–endoplasmic reticulum interface and serve as a platform to trigger apoptosis, although apoptosis and fission are separable [51] . However, our present work reveals that Fis1 is required for mitochondrial fission in cardiomyocytes. In addition to Fis1, we also observed an alteration of other mitochondrial fission-related factors, including MFF and Drp1, in response to anoxic treatment. The relationship between Fis1 and these factors in the apoptotic pathway of anoxia needs to be determined in future study. More than 800 miRNAs have been identified. Accordingly, it can be speculated that the identification of miRNAs that regulate proteins controlling mitochondrial fusion and fission may fill in the gap between unknown aspects of cell biology and the pathogenesis of diseases. Mitochondrial staining and analysis of mitochondrial fission Mitochondrial staining was carried out as we and others described with modifications [3] , [52] . Briefly, cells were plated onto the coverslips coated with 0.01% poly- L -lysine. After treatment, they were stained for 20 min with 0.02 μM MitoTracker Red CMXRos (Molecular Probes). Mitochondria were imaged using a laser-scanning confocal microscope (Zeiss LSM510 META). Generation of transgenic and KO mice For creating caFoxo3a transgenic mice, human caFoxo3a was obtained as we described [42] , and cloned to the vector pαMHC-clone26 (kindly provided by Dr Zhongzhou Yang) under the control of the α-myosin heavy chain (α-MHC) promoter. The primers used to generate caFoxo3a include, forward primer: 5′-ATGGCAGAGGCACCGGCTTCC-3′; reverse primer: 5′-TCAGCCTGGCACCCAGCTCTGAG-3′. Microinjection was performed following standard protocols. The primers for genotyping caFoxo3a transgenic mice include, forward primer in the α-MHC promoter, 5′-TGCCCAGCTGCCCGGCACTCT-3′; the reverse primer in the Foxo3a cDNA, 5′-CGGCCTTTGCAGGGGCCACG-3′. To generate miR-484 transgenic mice, a 425-bp DNA fragment containing murine miR-484 was cloned to the vector pαMHC-clone26 under the control of an α-MHC promoter. The primers used to generate miR-484 include, forward primer: 5′-CCAGTCGCTTCCTCCAGTAGC-3′; reverse primer: 5′-TTCTCTCCTTAGTCCTCGCTC-3′. The primers for genotyping miR-484 transgenic mice include forward primer in the α-MHC promoter, 5′-CAGAAATGACAGACAGATCCCTCC-3′; the reverse primer in the miR-484 DNA, 5′-AGTTCTTCGCCTGGAAGATCC-3′. Foxo3a KO mice were purchased from Mutant Mouse Regional Resource Center, USA. Foxo3a +/− mice were interbred to give KO mice (Foxo3a −/− ), which were used for further studies. Mice were genotyped by multiplex PCR (primers and conditions are available from Mutant Mouse Regional Resource Center, USA). All experiments were performed on Foxo3a −/− mice and their wild-type littermates (Foxo3a +/+ ). The animal experiments were performed according to the protocols approved by the Institute Animal Care Committee. miR-484 promoter and miRNA response element of miR-484 The miR-484 promoter region was amplified from rat genomic DNA to generate wild-type promoter. The forward primer was 5′-ATGATAGGGTGAGTGGAGAATGGTT-3′. The reverse primer was 5′-GAGAAGCTGAGGAAGGGTACGAAGT-3′. The PCR product was cloned into the vector pGL4.17 (Promega). The introduction of mutations in the putative Foxo3a-binding site in the wild-type fragment (−2,605 to −2,599 wild-type: 5′-GTAAACA-3′, the mutant: 5′-GCGGGCA-3′) was generated using QuikChange II XL Site-Directed Mutagenesis Kit (Stratagene). The construct was sequenced to check that only the desired mutations had been introduced. The miR-484 MREs were cloned into the region before luciferase translation stop code in the pGL3 luciferase vector (Promega). To test whether the target site is functional, we constructed eight mutants of MRE-1, in which the introduced mutations would result in no amino acid changes to the Fis1 protein. Quantitative real-time PCR Stem-loop quantitative real-time PCR (qRT–PCR) for mature miR-484 was performed as described [53] on an Applied Biosystems ABI Prism 7000 sequence detection system. Total RNA was extracted using Trizol reagent. After DNAse I (Takara, Japan) treatment, RNA was reverse transcribed with reverse transcriptase (ReverTra Ace, Toyobo). The levels of miR-484 analysed by qRT–PCR were normalized to that of U6. The U6 primers were forward: 5′-GCTTCGGCAGCACATATACTAA-3′; reverse: 5′-AACGCTTCACGAATTTGCGT-3′. ChIP assay ChIP assay was performed as we and others described with modifications [54] , [55] . In brief, cells (0.5×10 7 ) were washed with PBS and incubated for 10 min with 1% formaldehyde at room temperature. The cross-linking was quenched with 0.1 M glycine for 5 min. Cells were washed twice with PBS and lysed for 1 h at 4 °C in a lysis buffer. The cell lysates were sonicated into chromatin fragments with an average length of 500–800 bp as assessed by agarose gel electrophoresis. The samples were precleared with Protein-A agarose (Roche) for 1 h at 4 °C on a rocking platform, and 5 μg specific antibodies were added and rocked for overnight at 4 °C. Immunoprecipitates were captured with 10% (vol/vol) Protein-A agarose for 4 h. Before use, Protein-A agarose was blocked twice at 4 °C with salmon sperm DNA (1 μg ml −1 ), which had been sheared to a 500-bp length, and bovine serum albumin (1 μg ml −1 ) overnight. The final ChIP DNAs were then used as templates in qPCR reactions, using primers that encompass Foxo3a-binding site of the rat miR-484 promoter. The oligonucleotides were as follows: forward: 5′-CAGTCTCTCAAATGCTGAGAC-3′; reverse: 5′-GTTTAAGAACACTTTCTCAAG-3′. The specificity of the PCR amplification was confirmed by agarose gel electrophoresis. Preparation of subcellular fractions and immunoblot Subcellular fractions were prepared as we described [56] . In brief, cells were washed twice with PBS and the pellet was suspended in 0.2 ml of buffer A (20 mM HEPES (4-(2-hydroxyethyl)-1-piperazineethanesulfonic acid) pH 7.5, 10 mM KCl, 1.5 mM MgCl 2 , 1 mM ethylene glycol tetraacetic acid, 1 mM EDTA, 1 mM dithiothreitol, 0.1 mM phenylmethanesulfonylfluoride, 250 mM sucrose) containing a protease inhibitor cocktail. The cells were homogenized by 12 strokes in a Dounce homogenizer. The homogenates were centrifuged twice at 750 g for 5 min at 4 °C to collect nuclei and debris. The supernatants were centrifuged at 10,000 g for 15 min at 4 °C to collect mitochondria-enriched heavy membrane pellet. The resulting supernatants were centrifuged to yield cytosolic fractions. Immunoblot was carried out as we previously described [54] . Briefly, cells were lysed for 1 h at 4 °C in a lysis buffer (20 mmol l −1 Tris pH 7.5, 2 mmol l −1 EDTA, 3 mmol l −1 ethylene glycol tetraacetic acid, 2 mmol l −1 dithiothreitol, 250 mmol l −1 sucrose, 0.1 mmol l −1 phenylmethylsulfonyl fluoride, 1% Triton X-100) containing a protease inhibitor cocktail. Samples were subjected to 12% SDS–polyacrylamide gel electrophoresis and transferred to nitrocellulose membranes. Equal protein loading was controlled by Ponceau Red staining of membranes. Blots were probed using the primary antibodies. The antibodies to Fis1, Tom20, tubulin, actin, catalase and Mfn-1 were from Santa Cruz Biotechnology. The antibody to Foxo3a was from Cell Signaling. The antibodies to Drp1, cytochrome c and OPA1 were from BD Biosciences. The antibodies to Mfn-2, MFF and cytochrome oxidase subunit IV were from Abcam. After washing four times with PBS Tween-20, the horseradish peroxidase-conjugated secondary antibodies were added. Antigen–antibody complexes were visualized by enhanced chemiluminescence. The films were densitometrically scanned using NIH ImageJ. The ratios of the desired proteins to the particular loading controls were calculated, and the ratios of controls were assigned a value of one. Luciferase assay The mir-484 promoter luciferase assay was performed as we described [41] . Briefly, cells were seeded in 24-well plates. They were transfected with the luciferase constructs using the Lipofectamine 2000 (Invitrogen). Each well contains 0.2 μg luciferase reporter plasmids, 2.5 ng Renilla luciferase plasmids as the internal control. After transfection for 24 h, cells were exposed to anoxia and harvested at the indicated time after anoxia for the detection of luciferase activity, using the Dual Luciferase Reporter Assay kit (Promega) according to the manufacturer's instructions. A volume of 20 μl of protein extracts were analysed in a luminometer. Firefly luciferase activities were normalized to Renilla luciferase activity. Luciferase assays of Fis1 CDS and MREs were performed as we described elsewhere with modifications [41] . Cells were co-transfected with the luciferase constructs of 200 ng per well, along with the plasmid constructs of miR-484 or miR-484 control, miR-484 mimic or mimic-negative control, using Lipofectamine 2000 (Invitrogen). pGL3 vector served as a control. At 48 h after transfection, cells were lysed and luciferase activity was measured. Target protector preparation and transfection Target protector was designed and named as others and we described [40] , [41] . In brief, Fis1-TP miR-484 sequence is 5′-TCAAACTGCGTGCTCTTGGACACAG-3′. Fis1-TP control sequence is 5′-CCTCTTACCTCAGTTACAATTTATA-3′. They were synthesized by Gene Tools, and transfected into the cells using the Endo-Porter kit (Gene Tools) according to the kit's instructions. Analysis of mitochondrial connectivity Mitochondrial connectivity was analysed by fluorescence recovery after photobleaching as previously described [57] , [58] . In brief, cardiomyocytes were transfected with mitochondrial matrix-targeted GFP (pAcGFP1-mito, Clontech) using the FuGENE transfection reagent (Roche). The regions of interest were imaged at randomly chosen perinuclear regions of the cytoplasm that contained mitochondria, using an LSM 510 confocal microscope before and after photobleaching at 100% power with 488 nm laser. Scans were taken in 1 s intervals for a total of 60 images over 60 s. The fluorescence intensity in imaged ROIs was digitized with LSM 510 software (Zeiss MicroImaging). Fluorescence recovery was represented as a fraction of initial fluorescence after normalization to both non-specific photobleaching and background. Each fluorescence recovery after photobleaching curve represents the average of 30 measurements representative of results obtained in three separate experiments. Statistical analysis The results are expressed as mean±s.e.m. of at least three independent experiments. The statistical comparison among different groups was performed by one-way analysis of variance. The comparison between two groups was evaluated by Student's t -test. P <0.05 was considered statistically significant. How to cite this article: Wang K. et al . miR-484 regulates mitochondrial network through targeting Fis1. Nat. Commun. 3:781 doi: 10.1038/ncomms1770 (2012).